High mobility emissive organic semiconductor The integration of high charge carrier mobility and high luminescence in an organic semiconductor is challenging. However, there is need of such materials for organic light-emitting transistors and organic electrically pumped lasers. Here we show a novel organic semiconductor, 2,6-diphenylanthracene (DPA), which exhibits not only high emission with single crystal absolute florescence quantum yield of 41.2% but also high charge carrier mobility with single crystal mobility of 34 cm 2 V −1 s −1 . Organic light-emitting diodes (OLEDs) based on DPA give pure blue emission with brightness up to 6,627 cd m −2 and turn-on voltage of 2.8 V. 2,6-Diphenylanthracene OLED arrays are successfully driven by DPA field-effect transistor arrays, demonstrating that DPA is a high mobility emissive organic semiconductor with potential in organic optoelectronics. The achievement of organic semiconductors with both high mobility and strong fluorescence emission remains a challenge. High mobility requires molecules which pack densely and periodically, while serious fluorescence quenching typically occurs when fluorescent materials begin to aggregate (aggregation-induced quenching (AIQ)) [1] , [2] , [3] . Indeed, classical materials with strong fluorescent emission always exhibit low mobility [4] , [5] , [6] , [7] , for example, tris(8-hydroxyquinoline) aluminium (ALQ) [6] and phenylenevinylene-based polymers [7] with mobility only 10 −6 –10 −5 cm 2 V −1 s −1 , and benchmark organic semiconductors with high mobility demonstrate very weak emission [8] , [9] , [10] , [11] , for example, rubrene [10] exhibits a quantum yield <1% in crystalline state and pentacene [11] shows very weak fluorescence in the solid state. However, organic semiconductors with high mobility and strong fluorescence are necessary for the achievement of high efficiency organic light-emitting transistors (OLETs) [12] , [13] , [14] and electrically pumped organic lasers [15] , [16] . Here, we demonstrate a high mobility organic semiconductor (2,6-diphenylanthracene, DPA) with strong emission: for single crystals, mobilities as high as 34 cm 2 V −1 s −1 and photoluminescence quantum yield (PLQY) of 41.2% are obtained. OLEDs fabricated from this material give pure blue emission with brightness up to 6,627 cd m −2 with a turn-on voltage at 2.8 V. Moreover, organic light-emitting diode (OLED) arrays of this compound can be driven by organic field-effect transistors (OFETs) fabricated with DPA. For the first time, we see the possibility of integration of optoelectronic devices based on the same organic semiconductor. The design synthesis and characterization of DPA In the absence of significant intermolecular interactions (for example, in dilute solutions or when conjugated compounds are incorporated at very dilute concentrations in inert matrices), the radiative decay of these excitations are dominated by Kasha’s rule, and the luminescence efficiency is relatively high [1] , [2] . However, strong intermolecular interactions, for example, π–π co-facial stacking (H-aggregates), will cause the splitting of the lowest excited state (characterized by a non-emissive combination of the transition dipole moments of the individual molecule) resulting in optically forbidden transition to the ground state (AIQ). Thus, the luminescence is dramatically quenched ( Supplementary Fig. 1 ) [17] . Therefore, the challenge for high mobility emissive organic semiconductors is how to balance intermolecular packing (for efficient charge transport) and non-radiative energy transfer (for efficient emission). A novel compound, DPA ( Fig. 1a ), was designed and synthesized facilely with yield over 85% ( Supplementary Fig. 2 ). The rational design takes into the consideration (i) the strong fluorescence of anthracene as the core, (ii) the phenyl groups at 2-, 6- positions of anthracene core are used to extend the molecular π conjugation and tune the molecular packing. Indeed, the powder of DPA gives strong blue emission under UV light ( Fig. 1b ) with PLQY of 48.4% measured in a calibrated integrating sphere [18] . The high absolute quantum efficiency provides direct visual evidence of the strong emission of this compound. 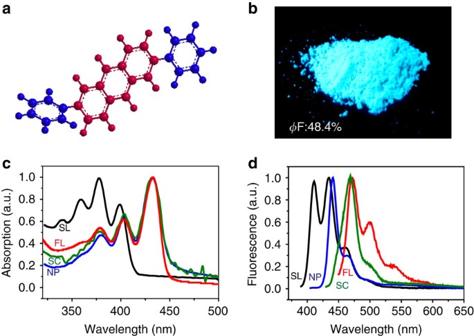Figure 1: Molecular structure of DPA and its corresponding absorption and emission features. (a) Molecular structure of DPA. (b) The powder of DPA gives strong blue emission under UV light with absolute fluorescent quantum yield up to 48.4%. (c,d) UV–vis and fluorescent spectra of DPA monomers in diluted solution (SL, black line), DPA nanoparticles in a THF:H2O=1:9 (v/v) mixture (NP, blue line), single crystals grown by PVT technique (SC, green line) and its vacuum-deposited thin film (FL, red line). Figure 1: Molecular structure of DPA and its corresponding absorption and emission features. ( a ) Molecular structure of DPA. ( b ) The powder of DPA gives strong blue emission under UV light with absolute fluorescent quantum yield up to 48.4%. ( c , d ) UV–vis and fluorescent spectra of DPA monomers in diluted solution (SL, black line), DPA nanoparticles in a THF:H 2 O=1:9 (v/v) mixture (NP, blue line), single crystals grown by PVT technique (SC, green line) and its vacuum-deposited thin film (FL, red line). Full size image To uncover the aggregation states of DPA solids, UV–vis and fluorescence measurements were conducted on DPA in different morphologies, including diluted solutions (10 μM) in tetrahydrofuran (THF), nanoparticles dispersed in a THF:H 2 O=1:9 (v/v) mixture, single crystals grown by physical vapour transport (PVT) technique [19] and vacuum-deposited thin films on a quartz plate. The use of nanoparticles is beneficial for determination of aggregation state of chromophores [20] , [21] , [22] . Here we included UV–vis and PL spectra of DPA nanoparticles for comparison. As shown in Fig. 1c,d , the lowest 0→0 transition of DPA in diluted solution appears at 398 nm as a sharp absorption peak along with the 0→1 and 0→2 transitions at 377 and 360 nm ( Fig. 1c , black line). The emission maximum of the DPA in solution ( Fig. 1d , black line) appears at 408 nm, yielding a Stokes shift of about 615.8 cm −1 . In comparison with DPA solution, the absorption and emission spectra of DPA nanoparticles demonstrate an obvious bathochromic shift with the maximum absorption peaks at 433 nm and the maximum emission peaks at 441 nm, respectively. The calculated Stokes shift for DPA nanoparticles in solution is ∼ 419.0 cm −1 , that is, much smaller than that of DPA in dilute solution (615.8 cm −1 ). As for single crystals and thin films, larger bathochromic shifts as compared with nanoaggregates are observed in the fluorescent spectra, and the maximum emission peaks are at 468 and 472 nm, respectively. Note that the absorption and emission spectra exhibit distinct vibronic sidebands. The 0–0 peaks are much stronger than the corresponding 0–1 or 0–2 transitions in solid states. The increased ratio of the 0–0 vibronic peak intensities compared with the 0–1 and 0–2 peaks in solid states suggests the formation of J-aggregates of DPA [23] which thereby minimize the fluorescence quenching in the solid state. Strong blue emission ( Fig. 2a ) is observed from the crystals and high PLQY of 41.2%. X-ray diffraction (XRD) patterns of DPA single crystals ( Supplementary Fig. 3 ) show strong and sharp diffraction peaks, demonstrating the high quality of the crystals. Single crystal X-ray crystallographic results (crystal size: ∼ 0.20 mm × 0.20 mm × 0.10 mm) demonstrate that DPA belongs to the P2(1)/c space group with crystal parameters of a =17.973(8) Å, b =7.352(3) Å, c =6.245(3) Å and β =90.646(9)°. Reflections of XRD results are indexed to be ( h00 ) peaks according to the single crystal structure, which implies that the ( h00 ) crystal plane is parallel to the surface of the substrate. Transmission electron microscopic (TEM) images of an individual hexagonal crystal and its corresponding selected area electron diffraction (SAED) pattern are shown in Fig. 2b,c . The SAED pattern is indexed with the lattice parameters obtained from bulk crystal: a =17.973(8) Å, b =7.352(3) Å, c =6.245(3) Å. The crystal facets could be indexed directly according to the law of constancy of interfacial angles from the regular hexagonal single crystals. The sharp diffraction peaks, clear edges and well assigned diffraction spots indicate the high quality of the crystals. 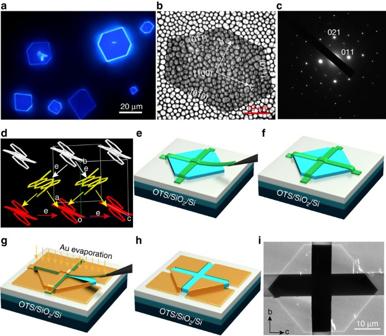Figure 2: DPA crystal features and device fabrication. (a) DPA crystals produced by PVT under UV light, the hexagonal crystals giving strong blue emissions. (b,c) Transmission electron microscopic image of individual DPA hexagonal crystal and its corresponding SAED pattern. (d) Charge transport alongbandcaxes in DPA crystal. (e–h) Fabrication of device based on individual micrometre-sized single crystal by `organic ribbon mask' technique on n-doped Si substrate with 300 nm SiO2and OTS monolayer. (i) An SEM image of an example transistor fabricated by the ‘organic ribbon mask’ technique. Figure 2: DPA crystal features and device fabrication. ( a ) DPA crystals produced by PVT under UV light, the hexagonal crystals giving strong blue emissions. ( b , c ) Transmission electron microscopic image of individual DPA hexagonal crystal and its corresponding SAED pattern. ( d ) Charge transport along b and c axes in DPA crystal. ( e – h ) Fabrication of device based on individual micrometre-sized single crystal by `organic ribbon mask' technique on n-doped Si substrate with 300 nm SiO 2 and OTS monolayer. ( i ) An SEM image of an example transistor fabricated by the ‘organic ribbon mask’ technique. Full size image Based on the structural information of the single crystals, the anthracene core of the DPA molecule is flat while the substituted phenyls are slightly out of the plane of conjugation with a torsion angle of 20.05° ( Supplementary Fig. 4a ). In crystal, DPA molecules adopt a herringbone packing motif as J-aggregates ( Fig. 2d and Supplementary Fig. 4b,c ) which effectively minimize the quenching of the DPA fluorescence in the solid state [17] , [24] , [25] . More detailed structure analysis demonstrates that the transition dipole moment is identified to be nearly parallel to the long axis of DPA molecule, which results in the bright edge emission of crystals ( Supplementary Fig. 5 ). In addition, multi- and strong intermolecular C–H–π interactions (with intermolecular distance only 2.84–2.86 Å) are observed between neighbouring DPA molecules ( Supplementary Fig. 6 ). Assuming one molecule accepts a charge, it could transfer the accepted charge to its near two neighbours, and then to other neighbours quickly, finally forming a two-dimensional network of charge transport ( Fig. 2d and Supplementary Fig. 7 ) [26] , [27] . These features are consistent with efficient charge transport and high mobility. DPA single crystal field-effect transistors To evaluate the charge transport properties of DPA, bottom-gate top-contact transistors based on individual DPA micrometre-sized crystals are fabricated with a ‘ribbon-mask-technique’ [28] , [29] based on octadecyltrichlorosilane (OTS)-treated Si/SiO 2 (300 nm) substrates as shown in Fig. 2e–h . First, hexagonal single crystals of DPA are deposited on the substrate by PVT ( Fig. 2e ). Second, micrometre or sub-micrometre organic ribbons prepared in advance are used as the mask. An individual organic ribbon is peeled off and put directly on a pre-deposited DPA crystal, and then another organic ribbon is laminated over the previous one at 90° ( Fig. 2f ). Third, Au is vacuum-deposited on the masked single crystal ( Fig. 2g ). Finally, the transistor with four crossed electrodes on an individual hexagonal crystal is obtained after the organic mask-ribbons are peeled off ( Fig. 2h ) (more details on device fabrication included in Methods). An example device based on an individual DPA crystal with four electrodes along b and c axes is shown in Fig. 2i . Transistors are measured on a Keithley 4200 SCS and Micromanipulator 6150 probe station with a high-resolution microscope (magnification at × 40–200) (in air and at room temperature) and the mobility is extracted from the equation of I DS =( W /2 L ) C i μ ( V G − V T ) 2 . The typical transfer and output characteristics are shown in Fig. 3a–c along the b axis and Fig. 3d–f along the c axis. Totally, 100 devices are examined, and over 95% devices exhibit mobility >10 cm 2 V −1 s −1 along b axis ( Fig. 3c ) with the maximum mobility up to 34 cm 2 V −1 s −1 , while along c axis only 75% devices demonstrate mobility over 10 cm 2 V −1 s −1 with the maximum mobility up to 23 cm 2 V −1 s −1 ( Fig. 3f ). We estimated 4.5 cm 2 V −1 s −1 for the linear mobility based on the data from Fig. 3a using 16.5 μm for the channel length and 3.3 μm for the channel width (assuming that the gate induced charge was confined to either the first two or the first four monolayers) indicating a relatively large contact resistance. 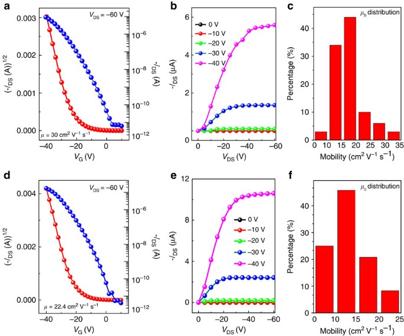Figure 3: Device performance of DPA single crystal transistors alongbandcaxes. (a,b) Typical transfer and output characteristics alongbaxis, which give mobility of 30 cm2V−1s−1with channel length of 16.5 μm and width of 3.3 μm. (c) Mobility distribution alongbaxis based on 56 devices. (d,e) Typical transfer and output characteristics alongcaxis, which give mobility of 22.4 cm2V−1s−1with channel length of 26.4 μm and width of 12.1 μm. (f) Mobility distribution alongcaxis based on 44 devices. Figure 3: Device performance of DPA single crystal transistors along b and c axes. ( a , b ) Typical transfer and output characteristics along b axis, which give mobility of 30 cm 2 V −1 s −1 with channel length of 16.5 μm and width of 3.3 μm. ( c ) Mobility distribution along b axis based on 56 devices. ( d , e ) Typical transfer and output characteristics along c axis, which give mobility of 22.4 cm 2 V −1 s −1 with channel length of 26.4 μm and width of 12.1 μm. ( f ) Mobility distribution along c axis based on 44 devices. Full size image The threshold voltage for the turn-on of the FETs is rather large, typically ∼ −20 V, indicating a high density of traps at the dielectric interface. Note also that there is a mismatch between the highest occupied molecular orbital (HOMO) energy level of DPA (5.6 eV) and the work function of gold (5.2 eV), which probably results in a relatively large contact resistance responsible for the initial curvature in the output data for V DS <−5 V as shown in Fig. 3 . Hence, further device optimization can be expected. The mobility anisotropy along different crystal directions is in the range of 1.3–1.5 along b and c axes ( Supplementary Fig. 8 ). DPA organic light-emitting diodes As an additional proof to confirm the high emission from this novel compound, OLEDs of DPA are fabricated as shown in Fig. 4a . A 40 nm N,N’-di-[(1-naphthyl)-N,N’-diphenyl]-1,1′-biphenyl)-4,4′- diamine (NPB) layer is inserted between indium tin oxide (ITO) and the emitting molecular layer (EML) of DPA films (30 or 40 nm) for energy level alignment to facilitate hole-injection and transport [30] . Here, DPA films are vacuum-deposited polycrystalline films composed of small crystalline domains as evidenced by their AFM images ( Supplementary Fig. 9a ), which have the same molecular packing structure and orientation as that of single crystals identified by the XRD results ( Supplementary Figs 3 and 9b ). For efficient electron-injection, LiF is adopted as the buffer layer. Moreover, considering the high mobility of DPA for efficient hole transport, another 30 nm 1,3,5-tri( p -pyrid-3-yl-phenyl)benzene (TMPYPB) is used as a hole-blocking and electron transport layer between LiF and DPA, because of the deep HOMO and low LUMO levels of TMPYPB. The energy-level diagram of the OLEDs is shown in Fig. 4b . The stepwise energy levels work efficiently for carrier injection and transport. Indeed, strong blue emission is observed from the DPA-based OLEDs as shown in Fig. 4c . A turn-on voltage of 2.8 V was achieved at the brightness of 1–10 cd m −2 and the maximum brightness was approaching 6,627 cd m −2 at 8.8 V when using 40 nm DPA as the active layer ( Fig. 4d ), which is higher than that of devices with 30 nm active layer ( Supplementary Fig. 9c,d ). 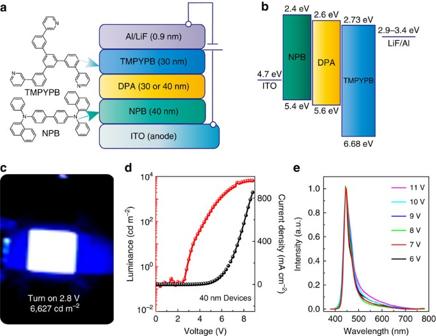Figure 4: OLEDs features of DPA. (a) OLEDs based on DPA with NPB, LiF and TMPYPB as buffer layers. (b) The energy-level diagram of OLEDs based on DPA. (c) Strong blue emission from OLEDs based on DPA (2 mm × 2 mm). (d) Current density-voltage-luminance characteristics of the OLEDs. (e) EL spectra operated at different voltages. Figure 4e shows the typical electroluminescence spectra (EL) of DPA-based OLEDs, which exhibits a sharp emission peak at 445 nm. There is no obvious shift under different voltages with the full-width at half-maximum of 35 nm. The OLED performance proves directly that DPA is an efficient blue emitter with low turn-on voltage and high brightness. Figure 4: OLEDs features of DPA. ( a ) OLEDs based on DPA with NPB, LiF and TMPYPB as buffer layers. ( b ) The energy-level diagram of OLEDs based on DPA. ( c ) Strong blue emission from OLEDs based on DPA (2 mm × 2 mm). ( d ) Current density-voltage-luminance characteristics of the OLEDs. ( e ) EL spectra operated at different voltages. Full size image DPA integrated optoelectronic arrays Integrated optoelectronic devices based on organic semiconductors is an essential goal for organic optoelectronic circuits [31] . One of the main obstacles is the lack of organic transistors with sufficiently high mobility and high ON–OFF ratio to achieve reasonable switching speeds in logic circuits [32] and to drive OLEDs. The different complex processes for the fabrication of OFETs and OLEDs also present a challenge to device integration. Here, we demonstrate the integration of our optoelectronic devices based on the same organic semiconductor, DPA. As an example, we choose a simple pixel-like configuration in which OFETs fabricated from the same material supply the current to drive the OLED arrays. The schematic representation of the circuit is shown in Fig. 5a,b ; and the OFET arrays driving the OLED arrays are shown in Fig. 5c . Note that the devices in Fig. 5 are thin film devices with measured mobility of approximately 3–4 cm 2 V −1 s −1 . When an OFET is switched on, the current flowed from the source electrode to the OLED cathode, and hence, the OLED could be switched on and off by the OFET gate voltage V G (for switching curves see Supplementary Fig. 10 ). A typical switched on OLED arrays are shown in Fig. 5d . By optimizing the device fabrication, at V G =−70 V, the OFET supplies a current density of ∼ 170 mA cm −2 to the OLED, resulting in a brightness at around ∼ 2,660 cd m −2 ( Supplementary Fig. 11 ). 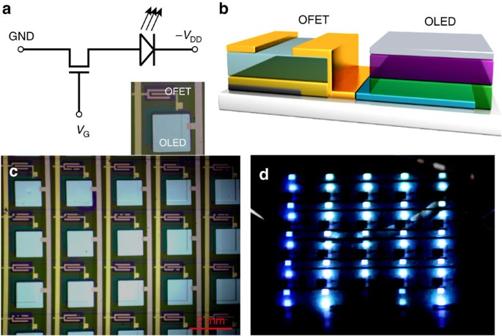Figure 5: Organic optoelectronic circuit of OFET driving OLED arrays based on DPA. (a,b) A configuration of OFETs driving OLED pixel, both OLED and OFET based on DPA. (c) Image of the OFET arrays driving OLED arrays. (d) Photo of the switched on DPA OLED arrays by DPA OFET arrays. GND, ground. Figure 5: Organic optoelectronic circuit of OFET driving OLED arrays based on DPA. ( a , b ) A configuration of OFETs driving OLED pixel, both OLED and OFET based on DPA. ( c ) Image of the OFET arrays driving OLED arrays. ( d ) Photo of the switched on DPA OLED arrays by DPA OFET arrays. GND, ground. Full size image For high performance OFETs, high mobility is essential, which requires molecules of organic semiconductors packing densely [26] , [27] . For example, Hu et al. found that molecules of α-titanylphthalocyanine (TiOPc) possess ultra close π-stacking structure with N6-N6 distance of 3.145 Å in convex pair and C9-C28 of 3.211 Å in concave pair, and hence thin film OFETs of α-TiOPc exhibited the highest mobility of 10 cm 2 V −1 s −1 and on/off ratio at 10 7 (ref. 33 ). Bao and Locklin et al. found that the reduced molecular packing distance of TIPS-pentacene from 3.33 to 3.08 Å by solution-shearing method could improve charge carrier mobility greatly from 0.8 to 4.6 cm 2 V −1 s −1 (ref. 34 ). However, generally, densely packed organic semiconductors will bring strong intermolecular coupling, which results in serious fluorescence quenching, so that benchmark organic semiconductors with high mobility demonstrate very weak [8] , [9] , [10] , [11] or even no emission [33] in the solid state. For OLEDs, organic semiconductor with strong emission is a pre-requirement in order to get high efficiency [3] , [4] , [5] , [6] . Moreover, it is necessary to limit the emission zone in the emissive layer and to have energy level alignment for well-balanced charge injection. Both are essential to provide efficient charge injection and carrier recombination for exciton formation and ultimately decay to the ground state with light emission. For the confinement of excitons in the active layer effectively, one needs charge carriers transporting not too fast in such thin active layer ( ∼ 100 nm), to provide enough time for exciton formation and decay, and hence low or moderate charge carrier mobility could meet the requirement. Hence, classical materials with strong fluorescent emission always exhibit low mobility [4] , [5] , [6] , [7] . The OLET is a novel concept transistor that emits light [12] , [13] , [14] . The OLET integrates light emission from the OLED and electrical switching by the OFET. Consequently, except excellent luminescence properties, ideal field-effect properties (for example, mobility) are also critically for an OLET. Moreover, by an elaborate design, the OLET could achieve minimum excitonic losses, efficient light confinement and high current density during operation while maintaining the quantum efficiency, and hence is considered to be a promising route toward realizing electrically driven organic laser [15] , [16] . Therefore, organic semiconductors that can meet the criteria of high mobility and strong emission are needed. According to exciton theory [35] , [36] , a fluorescent molecule is regarded as a dipole, and through the interaction of the two transition dipoles in a dimer, the excitonic state of the molecules splits into two levels. In an H-aggregate, the parallel dipoles (as the arrows in Supplementary Fig. 1 ) repel each other leading to a higher energy state, while the anti-parallel dipoles of a J-aggregate attract each other and lower the energy of that state. The syntropic dipoles get the lower energy state, while the reversed dipoles increase the energy of that state [37] . It is well known that, fluorescence is generated from the transition from the lowest excited state to the ground state [37] , [38] , for J-aggregates the lower exciton emission is allowed with a red-shifted fluorescence compared with the monomer, while the allowed transition in the H-aggregate is to the upper level with a blue-shifted fluorescence, vibrational relaxation from the upper level to the lower one explains the lower luminescence efficiency of H-aggregates [20] . Cornil et al. [17] , [39] proved that by adjusting the long axes of adjacent molecules to tune the molecular packing or to shift molecular packing from H-aggregation to J-aggregation works efficiently to prevent the quench of luminescence, because the dipole–dipole interactions in such molecular packing motifs are weakened. In our case, the non-planar DPA molecule (its anthracene core is flat while the substituted phenyls are slightly out of the conjugated plane with a torsion angle of 20.05°) indeed adopts J-aggregation, which works effectively to minimize the quenching of the fluorescence of DPA in solid state, so that the powder and crystal of DPA both give strong blue emission ( Figs 1b and 2a ). Meanwhile, multi-/strong intermolecular C–H–π interactions (with molecular distance only 2.84–2.86 Å) and compact molecular packing are observed in DPA crystals, that is, beneficial for efficient charge carrier transport. Assuming one molecule accepts a charge, it could transfer the accepted charge to its near two neighbours, and then to other neighbours quickly, finally forming a two-dimensional network of charge transport ( Supplementary Fig. 7 ). Indeed, DPA exhibits not only bright blue emission (quantum efficiency of 41.2%, electroluminescence >6,600 cd m −2 ), but also high hole mobility (up to 34 cm 2 V −1 s −1 ). This proves that the goal to obtain high mobility emissive organic semiconductor is accessible. Moreover, DPA OLED arrays can be driven successfully by DPA OFET arrays. This demonstrates the successful integration of optoelectronic devices based on the same organic semiconductor, indicating the potential of DPA in organic optoelectronics, especially planar integration. Material synthesis DPA is synthesized through three facile steps with yields over 85% ( Supplementary Fig. 2 ). 2,6-dihydroxyanthracene-9,10-dione was purchased from Sigma Aldrich and was used as received. Triethylamine and dichloromethane (dried by molecular sieve) were used for the esterification reaction. Tetrakis(triphenylphosphine)palladium(0) and trifluoromethanesulfonic anhydride was purchased from Strem Chemicals and were used as received. Nuclear magnetic resonance (NMR) spectra were recorded using a Bruker ADVANCE 400 NMR Spectrometer and 1 H NMR spectra were referenced to CDCl 3 (7.26 p.p.m.). Elemental analysis was carried out on Flash EA 1112 Elemental Analyser. AEI-MS50-MS spectrometer was used for molecular weight determination (more detailed synthesis information and characterizations see Supplementary Note 1 ). UV–vis and PL spectra measurement For Fig. 1b , the picture of DPA powder was taken under dark with a ultra-violet lamp shinning upon the compound with a wavelength of 365 nm. The UV–vis absorption spectra were measured with Hitachi (model U-3010) UV–vis spectrophotometer in a 1 cm quartz cell for solution samples. Nanoparticles of DPA were prepared by injecting 1.8 ml H 2 O to a stirring system of 0.2 ml 10 −4 M DPA solution in THF. Single crystals of DPA for UV–vis test were prepared by PVT technique with a sublimation temperature of 160 °C and a deposition temperature of 50–60 °C on quartz plate. And thin films of DPA samples for UV–vis test were fabricated by evaporation in high vacuum chamber on quartz plate under a pressure of 8 × 10 −4 Pa, and the deposition rates were monitored using a quartz oscillating crystal and controlled at 0.1 ∼ 0.2 Å s −1 . And photoluminescence spectra were recorded on a Perkin-Elmer LS 55 spectrofluorometer, the excitation wavelength was 390 nm for solution sample, 395 nm for nanoparticles and 430 nm for single crystals and thin films. For solid state sample, LabSphere, FluoroMax-4, HORIBA JobinYvon, PLQY software package were used. The PLQY was measured using the integrating sphere in combination with a commercial fluorimeter and a repeatable value of 48.4% was obtained for DPA powder and 41.2% for single crystals (grown on a circular quartz plate with a diameter of 1 cm). As for the thin films (PLQY, 19.5%) deposited on quartz plate, the PLQY is smaller than the crystals, which might be caused by the defects and grain boundaries in thin film state. Emission spectra including the scattering region of excitation light were measured for both blank and test samples, and these spectra were corrected with instrumental factors to calculate the quantum yield. For solution, 9,10-diphenyl anthracene was used as reference and a relative quantum yield of 62.7% was determined. FL picture of the crystals was recorded by laser scanning confocal microscope (Olympus FV-1000-IX81) under mercury lamp with a charge-coupled device (CCD) camera. Single crystal characterizations For single crystal data analysis, large crystals of DPA are grown from saturated solution in chloroform. The crystal analysis was performed on Rigaku Saturn724 CCD at 113(2) K using MoKα with diffraction radiation wavelength of 0.71073 Å and graphite as monochromator. For fluorescence property investigation and device fabrication, single crystals of DPA were grown by a physical vapour transport technique. Samples for laser scanning confocal microscope were grown on a 22 mm × 22 mm cover slip, and FL pictures of the crystals was recorded by laser scanning confocal microscope (Olympus FV-1000-IX81) under mercury lamp with a CCD camera. Samples for XRD characterization was grown on OTS/SiO 2 /Si substrates, considering the coverage of crystals on substrates, the substrate was turned four times with each time a different edge facing the sublimation source. X-ray diffraction measurement was performed in reflection mode at 40 kV and 200 mA with Cu Ka radiation using a 2 kW Rigaku D/max-2500 X-ray diffractometer. Samples for TEM test were prepared by scratching crystals from OTS/SiO 2 /Si and then transferred to copper grid with supporting carbon membrane. TEM and SAED measurements were carried out on a JEOL 2010 (Japan). Fabrication and measurement of DPA single-crystal OFETs The device fabrication of bottom-gate top-contact DPA single-crystal transistors followed the conventional procedures: (1) the heavily doped, n-type Si wafer containing a 300-nm-thick SiO 2 layer was used as substrate, which was successively cleaned with pure water, hot acetone, pure ethanol and oxygen plasma (about 15 s); (2) treatment of Si/SiO 2 wafer with OTS was then carried out by conventional vapour deposition method at a vacuum chamber (0.1 Pa) at 120 °C for 2.5 h; (3) single crystals of DPA were in-situ grown on OTS/SiO 2 /Si substrate by physical vapour transport in a horizontal furnace under 5 Pa, with DPA powder in the high temperature zone (160 °C) and the substrate at low temperature zone (50–60 °C) for OFET fabrication; (4) an ‘organic ribbon mask’ technique [29] was used to construct the devices with two perpendicular conducting channels based on an individual single crystal for anisotropic transport investigation. Under the assistance of micromanipulator 6150 probe station with a high-resolution microscope (magnification at × 40–200), micrometre or sub-micrometre organic ribbon prepared in advance on other substrates was peeled off and put directly on a pre-deposited DPA crystal with its direction just along the b or c axis, and then another organic ribbon was laminated over the previous one by a 90°, that is, c or b axes; (5) the substrate was transferred to a vacuum chamber and 50 nm gold was deposited on the masked single crystals; (6) the devices were finished by peeling off the ribbons. Organic field-effect transistor characteristics were obtained at room temperature in air on a Keithley 4200 SCS and Micromanipulator 6150 probe station and the mobility was extracted from the saturation region by using the equation of I DS =(W/2L)C i μ(V G −V T ) 2 . Fabrication and measurement of DPA OLEDs OLED devices were fabricated on ITO-coated glass substrate in a chamber with a pressure of 1 × 10 −4 Pa. Electroluminescence spectra characteristics of OLED devices were tested and analysed in air. J-V-L characteristics were measured using a computer-controlled Keithley 2400 Sourcemeter. The EL spectra were measured with a spectrascan PR650 photometer. Fabrication of integrated OFET-driving OLED arrays To construct the OFET-driving OLED arrays (AMOLED), we first fabricate OFETs based on ITO gate electrodes, which are patterned by photolithography (Suss MA6/BA6) and an etching process. Double layers of ALD-deposited HfO 2 (30 nm) and spin-coated polyamide acid (PAA) (300 nm) are used as gate dielectric with a capacitance of 20 nF cm −2 calculated through Keithley 590 CV analyser. Then, 50 nm DPA active layer was vacuum evaporated with 40 nm vacuum-deposited Au on top used as the source/drain electrodes. For OLED arrays, 40 or 20 nm semitransparent Au layer contacted the drain electrode of OFETs is vacuum-deposited on the PAA layer as the anode of the OLEDs. Subsequently, NPB/DPA/ TMPYPB/ LiF/ Al were vacuum thermally evaporated on the ITO anode in sequence. Finally, Cu was thermally evaporated on top for the data bus lines. The channel length and width of OFETs are 50 and 4,000 μm, respectively. The light-emitting area of OLED arrays is 400 × 400 μm 2 . AMOLEDs characteristics are tested and analysed in air. How to cite this article: Liu, J. et al. High mobility emissive organic semiconductor. Nat. Commun. 6:10032 doi: 10.1038/ncomms10032 (2015).